Atomic structure of amorphous shear bands in boron carbide Amorphous shear bands are the main deformation and failure mode of super-hard boron carbide subjected to shock loading and high pressures at room temperature. Nevertheless, the formation mechanisms of the amorphous shear bands remain a long-standing scientific curiosity mainly because of the lack of experimental structure information of the disordered shear bands, comprising light elements of carbon and boron only. Here we report the atomic structure of the amorphous shear bands in boron carbide characterized by state-of-the-art aberration-corrected transmission electron microscopy. Distorted icosahedra, displaced from the crystalline matrix, were observed in nano-sized amorphous bands that produce dislocation-like local shear strains. These experimental results provide direct experimental evidence that the formation of amorphous shear bands in boron carbide results from the disassembly of the icosahedra, driven by shear stresses. Covalent boron carbide (B 4 C) is one of the hardest materials known in nature, after diamond and cubic boron nitride. The unusual bonding of 12-atom icosahedra at polar sites with a three-atom chain in the rhombohedra unit cell of B 4 C forms a large open internal space and strong covalent bonds, giving rise to the unique properties of being extremely hard (~25–40 GPa in hardness) but very light (~2.5 g cm −3 in density) [1] , [2] , [3] , [4] , [5] , [6] , [7] . Therefore, B 4 C has been an important structural ceramic for the applications where both high strength and lightweight are required [6] , [7] . However, unlike other high performance ceramics, B 4 C displays an anomalous reduction in shear strength under pressures [8] , [9] , [10] , [11] . High-resolution electron microscopy of shock-loaded fragments revealed that the formation of nano-scale amorphous shear bands is responsible for the dramatic loss of shear strength at high pressures [12] . Diamond anvil cell experiments suggested that the local amorphization of B 4 C, associated with non-hydrostatic stress states, takes place during unloading from a pressure above a critical value of ~26 GPa [13] . In addition to shock loading and diamond anvil cell experiments, the amorphization has also been found when B 4 C is subjected to indentation and mechanical scratching [14] , [15] , [16] , [17] . These experimental observations demonstrated that the amorphous shear bands are the dominant deformation and failure modes of B 4 C at room temperature. On the basis of computer simulations and spectroscopic investigations, several controversial models have been proposed to explain the formation of amorphous shear bands in the super-hard material [1] , [13] , [14] , [16] , [17] , [18] , [19] , [20] , [21] . Nevertheless, the formation mechanisms of the amorphous shear bands still remain intensely debated owing to the lack of direct experimental observation with a sufficient spatial resolution to reveal the detailed structure of the amorphous bands. In this study, we employed the state-of-the-art spherical aberration (Cs) corrected scanning transmission electron microscopy (STEM) to characterize the structure of the deformation-induced amorphous shear bands in B 4 C. By utilizing the newly developed annular bright-field (ABF) STEM, which is advantageous for imaging light elements on atomic scale [22] , [23] , we provide direct evidence that the formation of amorphous shear bands results from the disassembly of the icosahedra in rhombohedral unit cells during shear deformation. Atomic structure of B 4 C Although the lattice images of the rhombohedra B 4 C can be readily achieved by conventional high-resolution transmission electron microscopy (HRTEM) [12] , [13] , detailed atomic structure of B 4 C, particularly 12-atom icosahedron and 3-atom chain in the unit cell, cannot be imaged because of the limited spatial resolution of the conventional HRTEM and the low contrast of the light elements of boron and carbon. In this study, we utilized ABF imaging technique using Cs-corrected STEM to achieve the ultrahigh spatial resolution of ~0.1 nm for the light elements. 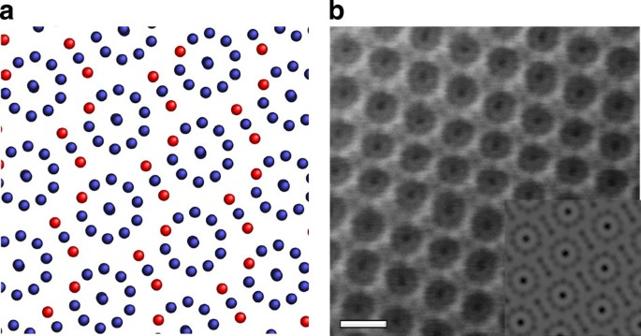Figure 1: Structure model and atomic image of B4C. (a) Projected structure model of the B4C along thedirection. Boron in blue and carbon in red colour. (b) Experimental ABF-STEM image of B4C along. Scale bar, 5 Å . The simulated ABF-STEM image is inserted at the bottom side. Figure 1a shows the structural model of B 4 C projected along a direction, which consists of B 11 C icosahedra and linear C–B–C atomic chains. The experimental ABF-STEM image ( Fig. 1b ) of crystalline B 4 C was taken from the thin region of a TEM specimen. Much more pronounced structural details, compared with the lattice images of HRTEM, can be observed. The ABF-STEM micrograph is consistent with the simulated ABF image as well (the inset of Fig. 1 ). The comparison between the experimental and simulated atomic images reveals the 12-atom icosahedra in the form of atomic rings and 3-atom chains as the dark lines linking the icosahedra. The ABF-STEM image is actually analogous to the direct projection of the structure model ( Fig. 1a ) along a same crystallographic direction. In fact, this is the first report of the atomic image of B 4 C, and, therefore, ABF-STEM is capable of detecting atomic-scale structure changes of B 4 C, which could not be achieved before. In this study, we employed this advanced imaging technique to probe the local atomic structure of amorphous shear bands in deformed B 4 C. Figure 1: Structure model and atomic image of B 4 C. ( a ) Projected structure model of the B 4 C along the direction. Boron in blue and carbon in red colour. ( b ) Experimental ABF-STEM image of B 4 C along . Scale bar, 5 Å . The simulated ABF-STEM image is inserted at the bottom side. Full size image Raman spectroscopy of amorphous B 4 C In this study, the amorphous B 4 C was introduced by a nanoindentation experiment [14] , [16] , [17] , [19] . 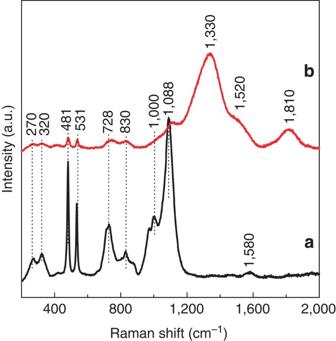Figure 2: Raman spectra of amorphous and crystalline B4C. (a) Representative Raman spectrum of pristine B4C; and (b) Raman spectrum taken from a residual indentation of microcrystalline B4C with 514 nm argon ion laser excitation. Figure 2 shows the representative Raman spectra acquired from the pristine and residual indented regions of B 4 C. The spectrum of the pristine B 4 C displays characteristic Raman peaks at 270, 320, 481, 531, 728, 830, 1,000 and 1,088 cm −1 assigned to crystalline B 4 C (refs 24 , 25 ), A weak band at 1,580 cm −1 has been attributed to the presence of a small fraction of graphitic carbon in sintered microcrystalline B 4 C (refs 7 , 16 ) ( Fig. 2a ). On indentation, the spectrum of the indented B 4 C reveals the most noticeable peak at 1,330 cm −1 , followed by a shoulder peak at 1,520 cm −1 and a broad peak at 1,810 cm −1 ( Fig. 2b ). These characteristic Raman bands indicate the formation of amorphous B 4 C caused by the indentation, in agreement with previous observations of amorphous B 4 C in single and polycrystalline B 4 C ceramics [14] , [16] , [17] , [19] . Figure 2: Raman spectra of amorphous and crystalline B 4 C. ( a ) Representative Raman spectrum of pristine B 4 C; and ( b ) Raman spectrum taken from a residual indentation of microcrystalline B 4 C with 514 nm argon ion laser excitation. Full size image ABF-STEM of amorphous shear bands To illustrate the structure of the indentation-induced amorphous B 4 C, the cross-sectional TEM specimen was sliced from a residual indent using a focused ion beam milling (FIB) technique [26] , [27] . The detailed process has been illustrated in Fig. 3 and described in the Methods section. Before cutting, an indentation region with the crystallographic direction was selected from the polycrystalline sample by using electron backscattered diffraction. Figure 4 shows the STEM images of the indentation region of B 4 C. Shear bands and micro-cracks, marked by the arrowheads, can be seen from the low magnification bright- and dark-field STEM images along the crystallographic direction ( Fig. 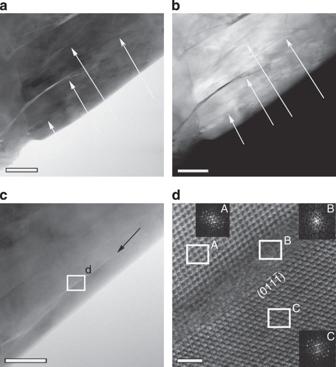Figure 4: Amorphous shear bands within the deformed area. (a) Low magnification bright-field and (b) dark-field STEM images of the deformed region. The shear bands and micro-cracks are indicated with arrowheads. Scale bar, 500 nm. (c) Bright-field STEM image of a zoom-in shear band with a length of ~200 nm. The black arrowhead shows the tip of the shear band. Scale bar, 50 nm. (d) ABF-STEM image of the shear band taken from the white-box region in (c). The high-resolution STEM image shows the amorphous structure of the shear band with a width of ~2 nm along thecrystallographic direction. Inset FFT patterns demonstrate the amorphous nature of the shear band. The slight mismatch in the orientation between the top and the bottom crystals can also be seen from the corresponding FFT patterns. Scale bar, 2 nm. 4a,b ), suggesting that extensive plastic deformation and damage take place underneath the indenter. In general, the micro-cracks show high contrast owing to complete separation by an open gap between two sides. Shear bands have much low contrast and usually have a width of ~2–3 nm and a length of ~100–200 nm ( Fig. 4c ). The zoom-in ABF-STEM image shows the loss of periodic crystalline structure within a shear band but voids and open gaps cannot be seen ( Fig. 4d ). The fast Fourier transform (FFT) pattern taken from the shear band displays a diffuse halo ring, confirming the occurrence of amorphization within the shear band ( Fig. 4d , inset B). In the crystalline substrate, the periodic icosahedron network can be well illustrated by the ABF-STEM image, implying that the sample fabricated by FIB is sufficiently thin to retain the high spatial resolution of ABF-STEM. The FFT patterns of the crystalline matrix display only the rhombohedral symmetry ( Fig. 4d , inset A and C). Therefore, except for shear bands and micro-cracks, the crystalline B 4 C matrix does not experience any structural transformation during the heavy indentation deformation. 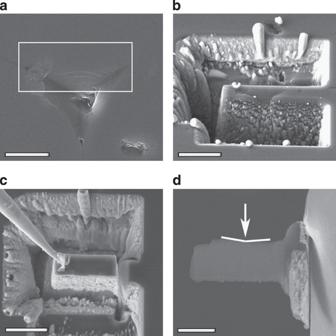From the FFT patterns of the crystalline matrix, it can be estimated that there is ~2° angular mismatch of the crystals between the two sides of the amorphous band, which is similar to the previous observations of amorphous shear bands in shock-loaded and diamond-anvil-cell-tested B 4 C (refs 12 , 13 ). Figure 3: Cross-sectional TEM sample preparation by FIB milling. (a) The selected region from the indentation impression (shown in white box) with the crystallographic direction of, estimated by electron backscatter diffraction. Scale bar, 5 μm. (b) Large trenches made around the selected region by FIB cutting. Scale bar, 10 μm. (c) A wedge-shaped TEM foil extracted by a microprobe. Scale bar, 10 μm. (d) Side view of the wedge-shaped specimen attached on the copper mesh by tungsten deposition (arrow showing indented impression). Scale bar, 5 μm. Figure 3: Cross-sectional TEM sample preparation by FIB milling. ( a ) The selected region from the indentation impression (shown in white box) with the crystallographic direction of , estimated by electron backscatter diffraction. Scale bar, 5 μm. ( b ) Large trenches made around the selected region by FIB cutting. Scale bar, 10 μm. ( c ) A wedge-shaped TEM foil extracted by a microprobe. Scale bar, 10 μm. ( d ) Side view of the wedge-shaped specimen attached on the copper mesh by tungsten deposition (arrow showing indented impression). Scale bar, 5 μm. Full size image Figure 4: Amorphous shear bands within the deformed area. ( a ) Low magnification bright-field and ( b ) dark-field STEM images of the deformed region. The shear bands and micro-cracks are indicated with arrowheads. Scale bar, 500 nm. ( c ) Bright-field STEM image of a zoom-in shear band with a length of ~200 nm. The black arrowhead shows the tip of the shear band. Scale bar, 50 nm. ( d ) ABF-STEM image of the shear band taken from the white-box region in ( c ). The high-resolution STEM image shows the amorphous structure of the shear band with a width of ~2 nm along the crystallographic direction. Inset FFT patterns demonstrate the amorphous nature of the shear band. The slight mismatch in the orientation between the top and the bottom crystals can also be seen from the corresponding FFT patterns. Scale bar, 2 nm. Full size image The detailed structure of the amorphous shear band shown in Fig. 4d is viewed from the direction close to of the crystal matrix. Because of the elastic strain field around the amorphous shear band, there is an orientation mismatch between the crystals residing at both sides of the amorphous band, as shown by the FFT patterns in Fig. 4d . Thus, it is difficult to align both crystals at their exact zone orientations simultaneously. The sample was first tilted to the orientation showing the sharpest crystal/amorphous interfaces, and, meanwhile, the crystal structure can be identified from both sides of the ~2 nm amorphous band ( Fig. 5a ). Deformed icosahedra with an imperfect ring shape are observed at the interface between the amorphous band and the crystal matrix, as shown in white circles ( Fig. 5a ). Although some icosahedra are significantly displaced from the lattice sites, others are hardly displaced, illustrating the gradual structure change from crystal to amorphous at the subnanoscale. As both crystals at the two sides of the amorphous band are not aligned at their exact zone orientation along this viewing direction, the defocus is set to image the crystal matrix and the structure of the amorphous band may be partially concealed as shown in Fig. 5a . To resolve the ambiguity of the amorphous band, the top-side crystal is perfectly aligned to projection ( Fig. 5b ). From this on-axis image, we can see that the icosahedral clusters are well unveiled, which are randomly distributed in the amorphous band. Moreover, the icosahedra loss their regular shape (shown in white circles). To further clarify the amorphous B 4 C structure, we have adjusted the bottom side ( Fig. 5a ) to the exact zone direction ( Fig. 5c ). From this view, we can readily detect the dangled and distorted icosahedral clusters in amorphous B 4 C region shown in white circles ( Fig. 5c ). Although the pronounced icosahedra can be recognized in the amorphous zone, their number density is apparently lower than that of the crystal matrix. This may be due to some icosahedra directly collapsing during the amorphization or tilting to orientations that cannot be imaged by ABF-STEM. 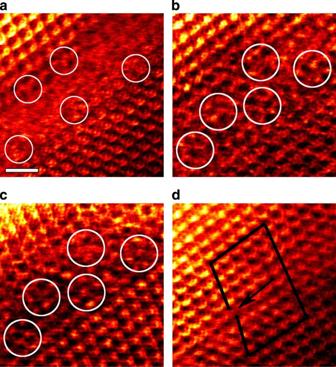Figure 5: ABF-STEM images of an amorphous shear band. (a) The image taken from slightly off-axis orientation from theB4C crystalline matrix. The displaced icosahedra at the amorphous/crystal interface are marked in white colour circles. (b,c) Retained icosahedra in the amorphous shear band imaged by on-axis ABF-STEM on either side of the crystal. The randomly distributed icosahedra in the amorphous band are denoted with white circles. (d) Shear displacement at the tip of the amorphous shear band. All images scale bar, 1 nm. Figure 5: ABF-STEM images of an amorphous shear band. ( a ) The image taken from slightly off-axis orientation from the B 4 C crystalline matrix. The displaced icosahedra at the amorphous/crystal interface are marked in white colour circles. ( b , c ) Retained icosahedra in the amorphous shear band imaged by on-axis ABF-STEM on either side of the crystal. The randomly distributed icosahedra in the amorphous band are denoted with white circles. ( d ) Shear displacement at the tip of the amorphous shear band. All images scale bar, 1 nm. Full size image Figure 5d is the ABF-STEM image taken from the tip region of the amorphous band, marked by the black arrowhead in Fig. 4c . The Burgers loop reveals the obvious lattice displacement along the amorphous band. The accumulated lattice strain at the tip of the amorphous band is analogous to a partial dislocation with a Burgers vector parallel to the shear band direction. Therefore, the amorphization of B 4 C gives rise to a shear displacement, equivalent to dislocation deformation in ductile crystals. On the other hand, this observation also demonstrates that the amorphization of B 4 C results from shear deformation. It is interesting to note that the amorphous shear bands, revealed by the ABF-STEM images, are along the crystal plane that is comprised of aligned three-atom chains ( Fig. 6 ). However, this plane is not the favourable dislocation slip plane of the rhombohedra B 4 C because the magnitude of the Burgers vector of dislocations on this plane is too large. Thus, dislocations and stacking faults cannot be formed on this plane under shear stress. Compared to the spherical icosahedra with closed atomic bonding, the three-atom chains are easier to deform (bending) and break when applied forces are not loaded along the chain direction [13] , [20] . Therefore, shear deformation preferentially takes place along this plane by the deformation and debonding of the three-atom chains when regular dislocation slip cannot be activated due to high Peierls stress at low temperatures. The occurrence of shearing along this plane may also be stimulated by the accumulation of thermal equilibrium point defects in the atomic chains [28] , which leads to the weakening of the chain structure. Likewise, multiple polyhedra of the chain structure (C–B–C, C–C–C, C–C–B and so on) [20] , together with the point defects (vacancies) in the chains, make this slip plane not have good long-range translational symmetry, and, hence, favourably form structure disorder when slip takes place. Moreover, the two identical debonding sites at the three-atom chains can also easily induce structure disorder when shear deformation takes place along this plane. 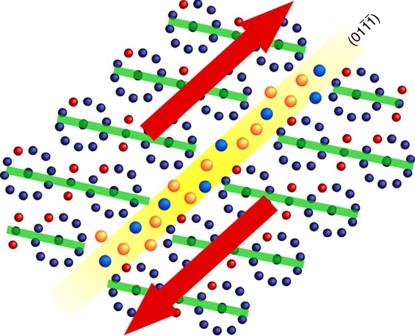Figure 6: Schematic of B4C amorphization by shear sliding along the plane. Shear-induced amorphization preferentially takes place along the B4C) plane that is comprises three-atom chains. Figure 6: Schematic of B 4 C amorphization by shear sliding along the plane. Shear-induced amorphization preferentially takes place along the B 4 C ) plane that is comprises three-atom chains. Full size image In summary, we have directly imaged the structure of amorphous shear bands in B 4 C by using the state-of-the-art ABF-STEM. The atomic-scale observations demonstrate the existence of retained icosahedra in nano-scale amorphous bands. Combining with crystallographic analysis, this study provides compelling experimental evidence on the underlying mechanisms of shear-induced amorphization of B 4 C. Material fabrication and nanoindentation experiment Fully dense microcrystalline boron carbide ceramic was consolidated by a hot pressing method [7] . The grain size of the sample ranges from 3–15 μm. A mirror-finish surface was prepared by careful polishing using diamond films. A series of indentations at a constant load of 2 N were performed with a dynamic ultra-micro-hardness tester (Shimadzu W201S) equipped with a Berkovich indenter. The mean hardness of the polycrystalline B 4 C was measured to be ~27 GPa and these indents were examined using a micro-Raman spectrometer (Renishaw, UK) with a 514 nm laser. The diameter of the laser spot was ~1 μm, which is ~4 to 5 times smaller than the dimension of residual impressions. TEM specimen preparation and characterization The cross-sectional TEM specimens of the indented B 4 C were prepared by a lift-out technique using a FIB system (JEOL JIB-4600F) ( Fig. 3 ). The indented B 4 C specimen was tilted to an angle of ~53° in the FIB system, and a large trench was made on either side of indented region using a high Ga + beam current with the accelerated voltage of 30 kV ( Fig. 3b ). After removing the remaining residual portion, the specimen was tilted back to its original position and a microprobe was attached on the top surface of the indent using tungsten deposition ( Fig. 3c ). The TEM foil was subsequently lifted out and attached onto a copper grid by tungsten deposition, followed by removal of microprobe tip from the TEM foil by Ga + beam cutting. Finally, the sample is thinned down to a thickness <50 nm by a low-energy ion beam ( Fig. 3d ). Before the TEM observations, the TEM sample was further gently milled by a Fishone 1040 Nanomill system to remove the damage layer on the sample surface without altering the specimen chemistry and structure. The microstructure of deformed samples was characterized with a TEM (TEM, JEOL JEM-2100F) with double Cs correctors. The ABF-STEM images were recorded by Gatan DF detector with the detector angle of ~11–23 mrad and point-to-point resolution 0.1 nm. ABF-STEM image simulations were performed by using a software package of Win HREM (HREM Research Inc). How to cite this article: Reddy, K.M. et al. Atomic structure of amorphous shear bands in boron carbide. Nat. Commun. 4:2483 doi: 10.1038/ncomms3483 (2013).